FGF signalling restricts haematopoietic stem cell specification via modulation of the BMP pathway Haematopoietic stem cells (HSCs) are produced during embryogenesis from the floor of the dorsal aorta. The localization of HSCs is dependent on the presence of instructive signals on the ventral side of the vessel. The nature of the extrinsic molecular signals that control the aortic haematopoietic niche is currently poorly understood. Here we demonstrate a novel requirement for FGF signalling in the specification of aortic haemogenic endothelium. Our results demonstrate that FGF signalling normally acts to repress BMP activity in the subaortic mesenchyme through transcriptional inhibition of bmp4 , as well as through activation of two BMP antagonists, noggin2 and gremlin1a . Taken together, these findings demonstrate a key role for FGF signalling in establishment of the developmental HSC niche via its regulation of BMP activity in the subaortic mesenchyme. These results should help inform strategies to recapitulate the development of HSCs in vitro from pluripotent precursors. Haematopoietic stem cells (HSCs) ultimately maintain all lineages of blood and immune cells throughout the lifetime of an organism. This feature underlies the long-term efficacy of bone marrow transplantation, frequently used as therapy for blood disorders including leukaemia. Immune incompatibility between donor and host, insufficient number of donors and the rarity of HSCs within many donor tissues have led to a search for alternative approaches to traditional HSC-based therapies. Recent breakthroughs using induced pluripotent stem cells have brought hope of in vitro derived, patient-specific HSCs, which could circumvent these issues. Despite decades of effort, it is not currently possible to generate bona fide HSCs from pluripotent precursors. The development of novel HSC-based therapeutics may thus depend on obtaining a more precise understanding of the native molecular events that occur in vivo during HSC formation. In all vertebrate animals examined, HSCs arise during embryogenesis from a specialized population of arterial cells localized in the ventral side of the dorsal aorta (DA) termed haemogenic endothelium [1] . This endothelial–haematopoietic transition [2] appears to exist only transiently, and is characterized by changes in gene expression and shape in ventral aortic endothelial cells as HSC precursors emerge and then enter circulation [2] , [3] , [4] , [5] , [6] . A prerequisite for HSC emergence appears to be the normal specification of arterial fate, most importantly proper formation of the DA. At the molecular level, arterial identity is governed by multiple extrinsic signals. In the zebrafish embryo, hedgehog signals from the notochord/floor plate regulate the expression of Vascular Endothelial Growth Factor A (VegfA) and calcitonin in the somites, which in turn regulate expression of Notch receptors in the DA [7] , [8] , [9] , [10] , [11] . Modulation of any of these signalling pathways alters arterial development and therefore HSC formation. Recent studies have demonstrated that HSC formation is disrupted by defects in the Wnt16 (ref. 12 ), VegfA [13] and bone morphogenetic protein 4 (Bmp4) (ref. 14 ) pathways without concomitant loss of aortic fate. Interestingly, each pathway regulates different steps of HSC development. In zebrafish, Wnt16 controls early HSC specification through its regulation of the somitic Notch ligand genes deltaC and deltaD , whose combined action is required for the Notch-dependent specification of HSCs, but not for arterial development [12] . More recently, it was confirmed in Xenopus that arterial fate and HSC emergence can be uncoupled based on VegfA isoforms. The short isoform controls arterial fate likely through Notch4, while HSC emergence depends on the medium/long isoforms and Notch1 (ref. 13 ). Finally, Bmp4 that is localized to the subaortic mesenchyme is responsible for the polarization of HSC formation from the ventral side of the DA [14] , [15] , [16] , [17] . Smad1, an intracellular activator of the BMP pathway, transactivates the runx1 promoter in vitro , suggesting that Bmp4 may act directly upstream of runx1 (ref. 18 ), which is required for the emergence of HSCs across vertebrate species [8] , [19] , [20] , [21] . Just before the onset of definitive haematopoiesis in zebrafish, the aortic region switches from a BMP repressive to activated environment [14] . The mechanism of this sudden change remains unknown. Interplay between BMP and fibroblast growth factor (FGF) signalling pathways has been described during organogenesis. In Xenopus , FGF and BMP signalling pathways intersect in the regulation of primitive erythropoiesis where FGF inhibits Bmp4-induced erythropoiesis through the control of gata2 (ref. 22 ). The repressive role of FGF in primitive blood is conserved across the vertebrates. For instance, in the chicken embryo, FGF signals through Fgfr2 to control erythrocyte differentiation by repressing gata1 expression in blood precursors [23] . In Xenopus , FGF was shown to act on the timing of primitive haematopoiesis by holding back the onset of the molecular programme that triggers primitive blood formation [24] . Finally, in zebrafish, primitive erythrocyte formation depends on Fgf21, which also governs erythromyeloid precursor development, likely in concert with Fgf1 (refs 23 , 25 , 26 ). While several studies have established that FGF signalling represses primitive blood formation, FGF signalling acts as a positive regulator of adult HSCs. Fgf1 (ref. 27 ) and Fgf2 (ref. 28 ) can expand ex vivo the number of transplantable HSCs. However, this effect seems to be limited to the short-term HSC compartment in vivo and it is accompanied by an alteration in the terminal differentiation of erythrocytes, B cells and myeloid cells [29] . More recently, the role of FGF signalling in steady state conditions has been challenged and seems to be mainly required to promote mobilization and proliferation of HSCs under stress-induced conditions [30] , [31] . FGF signalling appears to have multiple roles in blood development; however, its potential role in the emergence of HSCs has not been addressed. In this study, we have discovered a key repressive role for FGF signalling in HSC emergence through its regulation of the BMP pathway. Together with the data in the accompanying paper (Lee et al . ), which reveals an earlier positive role for FGF in programming the HSC lineage, these findings suggest that precise temporal inhibition as well as activation of FGF signalling may aid in vitro approaches to instruct HSC fate from pluripotent precursors. FGF signalling is a negative regulator of HSC formation To functionally test whether or not FGF signalling is required for definitive blood formation, we utilized transgenic zebrafish in which FGF signalling can be inducibly abrogated or enforced by heat-shock induction of a dominant-negative Fgfr1-EGFP fusion protein ( hsp70:dn-fgfr1-EGFP) [32] , [33] or a constitutively active Fgfr1 mutant protein ( hsp70:ca-fgfr1 ) [34] , respectively. This time-controlled approach allowed us to avoid mesoderm patterning defects induced by early FGF misexpression and subsequently target different developmental events according to their timing [35] . To identify temporal windows when FGF signalling is involved in HSC development, we initially targeted the early stage of arterial specification by inducing the hsp:dn-fgfr1 transgene at 17 h.p.f. (hours post fertilization, 15 somite stage). At this stage, primitive blood and endothelial cells are specified and the first sign of arterial specification is detectable in the endothelial precursors that are migrating from the lateral plate mesoderm to the midline [36] to form the primitive vascular cord [37] , [38] , [39] . Transgenic embryos were then sorted based on the expression of green fluorescent protein (GFP), and GFP-negative embryos were used as sibling controls. Following induction of hsp:dn-fgfr1 , definitive haematopoiesis initiated normally and there was no significant difference in runx1 expression between GFP+ and GFP− animals ( Supplementary Fig. 1A,B ). Interestingly, arterial and endothelial differentiations were unaffected, based on the normal expression of deltaC and kdrl , respectively ( Supplementary Fig. 1C–F ), suggesting that FGF signalling is not required for arterial differentiation or vascular development during the convergence of vascular precursor cells to the midline. To investigate possible later requirements for FGF signalling in HSC development, embryos were heat shocked at 20.5 h.p.f. (23 somite stage), just before runx1 expression along the aortic floor marks initiation of the definitive HSC programme. To verify loss of FGF signalling, we analysed the expression of pea3 , a direct transcriptional target [40] of FGF signalling. In embryos heat shocked at 20.5 h.p.f., pea3 expression decreased, and was accompanied by an increase in runx1 expression ( Fig. 1a,b,d,e ). At the stage when the heat shock was performed, the aortic region contains the precursors of the HSCs that will specifically express runx1 from 23 h.p.f., but also primitive blood that can be distinguished from HSC based on gata1 expression. The effect of the modulation of FGF signalling is restricted to the HSCs as shown by the absence of alteration of gata1 expression in transgenic embryos ( Supplementary Fig. 2A ). EMPs (erythromyeloid progenitor), bipotent precursors that arise in the posterior blood island [41] , are not affected on FGF modulation ( Supplementary Fig. 2A ). In converse experiments, where FGF signalling was enforced via 20.5 h.p.f. induction of the hsp:ca-fgf1 transgene, embryos exhibited embryo-wide upregulation of pea3 expression and a substantial decrease in runx1 expression along the aortic floor ( Fig. 1c,f ). Despite strong GFP expression at 5 h post heat shock (hpHS), hsp:dn-fgfr1 embryos displayed only a slight decrease in pea3 expression, leading to the conclusion that cellular turnover of the truncated receptor may outpace the turnover of GFP. To address this, pea3 expression was analysed in hsp:dn-fgfr1 embryos from 23 to 27 h.p.f. At 2 hpHS, pea3 was nearly absent in GFP+ embryos. Expression of pea3 gradually returned to normal around 6 hpHS ( Supplementary Fig. 2B ). Effects on runx1 expression followed this trend. Between 2 and 4 hpHS, a greater proportion of hsp:dn-fgfr1 embryos showed stronger upregulation of runx1 than when analysed between 5 and 6 hpHS ( Supplementary Fig. 2C ). The effects of Fgf modulation on runx1 expression were confirmed by quantitative PCR (qPCR) using complementary DNAs from the dissected trunks of hsp:dn-fgfr1 and hsp:ca-fgfr1 embryos ( Fig. 1g ). 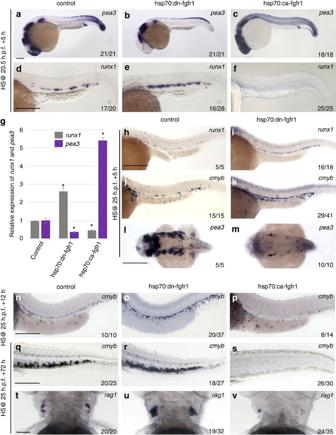Figure 1: FGF signalling represses HSC formation and maintenance. (a–f) Embryos were heat shocked at 20.5 h.p.f. and analysed at 26 h.p.f. (a–c)pea3expression is downregulated inhsp:dn-fgfr1(b) and upregulated inhsp70:ca-fgfr1embryos (c) compared with controls (a). (d–f) Aortic expression ofrunx1is enhanced inhsp70:dn-fgfr1(e) and depleted inhsp70:ca-fgfr1embryos (f) compared with controls (d). (g) Quantification ofrunx1andpea3mRNA expression in dissected trunks normalized toef1α. Expression of each gene was set to 1 in the control (mean±s.d.,n>3, *P<0.001, Student’st-test). (h–m) Embryos were heat shocked at 25 h.p.f. and analysed at 30 h.p.f. (h–i)runx1expression is increased inhsp70:dn-fgfr1embryos (i) compared with controls (h). Similar results are seen withcmybexpression in control (j) andhsp70:dn-fgfr1embryos (k). (l,m) Dorsal view ofpea3expression in the head shows downregulation ofpea3on depletion of FGF signalling. (n–v) Embryos were heat shocked at 25 h.p.f. and analysed 12 h and 72 hpHS. (n–p)cmybexpression is more intense in thehsp70:dn-fgfr1embryos (o) compared with control embryos (n). Conversely, embryos in which FGF signalling is increased display a drastic diminution ofcmybexpression (p). (r,q–s) Comparison ofcmybexpression in the CHT of heat shocked transgenic embryos and controls. The augmentation of HSC numbers detected at 26 h.p.f. on FGF modulation is maintained in the CHT of thehsp70:dn-fgfr1embryos while the CHT of thehsp70:ca-fgfr1embryos are devoid ofcmybcells. (t–v) Effect of FGF signal alteration on T cells. FGF ablation (u) or augmentation (v) has opposite effects onrag1+cells. Scale bars, 50 μm (a), 200 μm (d,h), 250 μm (l,n,q) and 50 μm (t). Figure 1: FGF signalling represses HSC formation and maintenance. ( a – f ) Embryos were heat shocked at 20.5 h.p.f. and analysed at 26 h.p.f. ( a – c ) pea3 expression is downregulated in hsp:dn-fgfr1 ( b ) and upregulated in hsp70:ca-fgfr1 embryos ( c ) compared with controls ( a ). ( d – f ) Aortic expression of runx1 is enhanced in hsp70:dn-fgfr1 ( e ) and depleted in hsp70:ca-fgfr1 embryos ( f ) compared with controls ( d ). ( g ) Quantification of runx1 and pea3 mRNA expression in dissected trunks normalized to ef1α . Expression of each gene was set to 1 in the control (mean±s.d., n >3, * P< 0.001, Student’s t -test). ( h – m ) Embryos were heat shocked at 25 h.p.f. and analysed at 30 h.p.f. ( h – i ) runx1 expression is increased in hsp70:dn-fgfr1 embryos ( i ) compared with controls ( h ). Similar results are seen with cmyb expression in control ( j ) and hsp70:dn-fgfr1 embryos ( k ). ( l , m ) Dorsal view of pea3 expression in the head shows downregulation of pea3 on depletion of FGF signalling. ( n – v ) Embryos were heat shocked at 25 h.p.f. and analysed 12 h and 72 hpHS. ( n – p ) cmyb expression is more intense in the hsp70:dn-fgfr1 embryos ( o ) compared with control embryos ( n ). Conversely, embryos in which FGF signalling is increased display a drastic diminution of cmyb expression ( p ). ( r , q – s ) Comparison of cmyb expression in the CHT of heat shocked transgenic embryos and controls. The augmentation of HSC numbers detected at 26 h.p.f. on FGF modulation is maintained in the CHT of the hsp70:dn-fgfr1 embryos while the CHT of the hsp70:ca-fgfr1 embryos are devoid of cmyb cells. ( t – v ) Effect of FGF signal alteration on T cells. FGF ablation ( u ) or augmentation ( v ) has opposite effects on rag1+ cells. Scale bars, 50 μm ( a ), 200 μm ( d , h ), 250 μm ( l , n , q ) and 50 μm ( t ). Full size image Before 26–27 h.p.f., the close proximity of primitive erythrocytes within the DA and posterior cardinal vein (PCV) to the floor of the DA [42] makes it difficult to distinguish them from emerging HSCs, since each lineage shares expression of early haematopoietic markers. We therefore shifted the heat-shock regimen to 25 h.p.f. and fixed at 30 h.p.f. By this time, erythroid precursors would have entered circulation, which allows visualization of the haemogenic endothelial marker cmyb by whole-mount in situ hybridization (WISH). Induced hsp70:dn-fgfr1 embryos showed elevated expression of both runx1 and cmyb in the DA ( Fig. 1h–k ; Supplementary Fig. 2D ) within the period during which the FGF transcriptional target pea3 is still downregulated ( Fig. 1l,m ). In mammals, HSCs leave the DA region quickly after their emergence to seed the fetal liver and the thymus. In zebrafish, a similar shift occurs: runx1+/cmyb+ cells migrate from the DA to the caudal haematopoietic tissue (CHT) and the thymus [43] , [44] , [45] . To ascertain whether the expanded pool of runx1+/cmyb+ cells are HSCs, FGF signalling was modulated at 25 h.p.f. and the effect on HSCs was monitored in the DA, the CHT and the thymus at 36 h.p.f. (25 h.p.f.+12 h), 3 (25 h.p.f.+48 h) and 4 days post fertilization (d.p.f.) (25 h.p.f.+72 h; Fig. 1n–v ; Supplementary Fig. 2E,F ). In induced hsp70:dn-fgfr1 embryos, cmyb expression is still expanded in the DA 12 hpHS ( Fig. 1n,o ). Conversely, embryos in which FGF signalling was enforced are devoid of cmyb cells in the DA ( Fig. 1n,p ). Similarly, at 48 and 72 hpHS, hsp70:dn-fgfr1 embryos showed a more robust expression of runx1 and cmyb in the CHT, while hsp70:ca-fgfr1 embryos showed a drastic decrease of the runx1+ and cmyb + cells ( Supplementary Fig. 2E ; Fig. 1q–s ). qPCR analysis of dissected CHT confirmed that runx1 , cmyb and CD41 levels of expression vary according to the modulation of FGF signalling ( Supplementary Fig. 2F ). T cells are thought to be the first functional derivatives of HSCs. They are first detected around 3 d.p.f. and by day 4, rag1 expression becomes robust in the thymus. The effect of FGF signalling modulation at 25 h.p.f. also affects the number of thymic rag1+ cells ( Fig. 1t–v ). Importantly, the increase in the number of rag1+ cells was observed only in hsp70:dn-fgfr1 embryos whose blood circulation was unaffected. Taken together, these results demonstrate that FGF signalling is important in the establishment of haemogenic endothelium, acting to repress the specification of HSC fate from the aortic floor. Fgf10a represses HSC formation by acting on fgfr2 and fgfr3 To identify the cell types that may mediate the effects of FGF signalling on HSC emergence, we examined localization of Fgf receptor expression at 20.5 h.p.f. and at 24 h.p.f. ( Supplementary Fig. 3 ). Fgfr1a , fgfr1b and fgfr4 were not detected in the tissues surrounding the DA at either time point ( Supplementary Fig. 3A–H,Q–T ). Fgfr2 showed strong expression in the pronephric ducts, the hypochord and the neural tube at 20.5 h.p.f. ( Supplementary Fig. 3I,J ). In contrast to fgfr2 , fgfr3 transcripts were detected in the somites at 20.5 h.p.f. ( Supplementary Fig. 3M,N ). At 24 h.p.f., fgfr3 is expressed throughout the trunk, whereas fgfr2 expression is restricted to the neural tube, the pronephric ducts, the hypochord and in cells surrounding the axial vasculature ( Supplementary Fig. 3K,L,O,P ). The localization of each receptor suggests that the effects of FGF modulation on HSC formation may act through fgfr2 and/or fgfr3. However, morpholino knockdown of these receptors failed to phenocopy the increase in runx1 and cmyb expression observed in the hsp70:dn-fgfr1 transgenic line. Loss of either receptor led to the absence of runx1 expression in the DA at 26 h.p.f. ( Supplementary Fig. 4 ). The discrepancy between the phenotype observed in morphants and that observed in hsp70:dn-fgfr1 embryos suggests that fgfr2 and fgfr3 may be required at earlier stages of mesoderm or vascular development. In zebrafish, 27 Fgf ligands have been identified [46] . At the stage of the heat shock, fgf10a is expressed throughout the trunk [47] , which made it a good candidate. To analyse its potential role in HSC specification, knockdown experiments were carried out using a splice-blocking morpholino ( Fig. 2 ). Our LOF (loss of function) experiments showed that depletion of fgf10a gives a similar phenotype to the phenotype observed in the hsp70:dn-fgfr1 embryos. At 30 h.p.f., in morphant embryos, runx1 and cmyb expressions are extended along the entire DA ( Fig. 2a–e ). 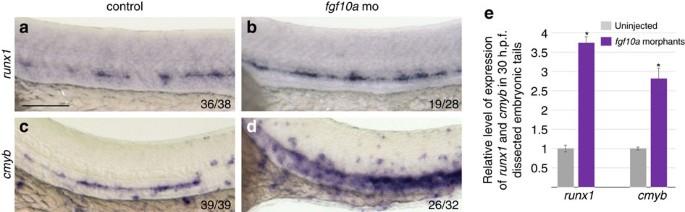Figure 2: Loss offgf10amimics the effect of FGF ablation. (a,b)runx1expression is expanded along the entire DA in the morphant embryos. Similarly, loss of Fgf10a significantly increases cmyb expression in the aortic region (c,d). Comparison of the relative levels of expression ofrunx1andcmybby qPCR in control and morphant embryos (e; mean±s.d.,n=3, *P<0.001, Student’st-test). Scale bar, 150 μm. Figure 2: Loss of fgf10a mimics the effect of FGF ablation. ( a , b ) runx1 expression is expanded along the entire DA in the morphant embryos. Similarly, loss of Fgf10a significantly increases cmyb expression in the aortic region ( c , d ). Comparison of the relative levels of expression of runx1 and cmyb by qPCR in control and morphant embryos ( e ; mean±s.d., n =3, * P< 0.001, Student’s t -test). Scale bar, 150 μm. Full size image Taken together, our results confirm that FGF signalling acts as a negative regulator of definitive haematopoiesis. This function is mediated by fgf10a, which likely signals through fgfr2 and/or fgfr3. FGF acts independently of the Notch and Vegf pathways In both mouse and zebrafish, Notch signalling is required for aortic and HSC specification [9] , [21] , [48] , [49] . As fgfr2 is expressed in the aortic region and fgfr3 in the somites, it is possible that the effects of FGF signalling on HSC emergence could be due in part to the effects on the Notch pathway. In zebrafish, enforced expression of the Notch intracellular domain (NICD) throughout the embryo is sufficient to generate an excess of HSCs [21] . Similarly in mice, genetic depletion of COUP-TFII, which normally represses Notch in the PCV, leads to the formation of ectopic haematopoietic clusters in the PCV [50] . We therefore investigated whether the modulation of HSC number observed in the DA following loss or gain of FGF signalling might be due to effects on the Notch pathway. Transgenic hsp70:dn-fgfr1 or hsp70:ca-fgfr1 embryos were heat shocked at 20.5 h.p.f., fixed at 25 h.p.f. and then assayed for Notch-related vascular and arterial gene markers by WISH ( Supplementary Fig. 5A–O ). Following either loss or gain of FGF function, the integrity of the vascular system was unaffected, as indicated by normal kdrl expression ( Supplementary Fig. 5A–C ). Aortic markers, including gridlock (a target of the Vegf pathway [9] ; Supplementary Fig. 3D–F ), notch1b ( Supplementary Fig. 5G–I ) deltaC ( Supplementary Fig. 5J–L ) and ephrinb2a (a target of the Notch pathway [48] ; Supplementary Fig. 5M–O ), were unchanged following modulation of FGF signalling. These results indicate that the effects of FGF signalling on HSC fate are not dependent on downstream Notch signalling events. To test the converse, that is, whether or not FGF signalling requirements are downstream of Notch, Notch signalling was blocked using N -[ N -3,5-difluorophenacetyl]- L -alanyl- S -phenylglycine Methyl Ester (DAPM), a small chemical inhibitor of NICD released from Notch receptors. If the increase in HSC number following FGF inhibition acts downstream of Notch, blockade of Notch signalling in the same temporal window as FGF inhibition should not prevent runx1 upregulation in the DA. In accord with this hypothesis, hsp70:dn-fgfr1 embryos treated with DAPM maintained strong expression of runx1 in the DA ( Supplementary Fig. 5P–U ). These results demonstrate that the increase in HSC number observed in absence of FGF signalling acts in a dominant manner with respect to loss of Notch signalling. Taken together, our studies on the interaction of Notch and FGF suggest that the effects of FGF on HSC fate either occur independently or downstream of the roles of the Notch/Vegf signalling axis during arterial development and HSC formation. FGF signalling does not affect dorsal polarization of the DA Since the increase in HSC marker expression in the DA is not a result of overactivation of the Vegf or Notch signalling pathways, we reasoned that it may be due to an increase in the number of runx1+ cells in the DA or the surrounding mesenchyme. We thus examined runx1 expression in transverse sections following induction of the hsp70:dn-fgfr1 transgene at 20.5 h.p.f. In wild-type (WT) controls, rare runx1 + cells were visible only in the floor of the DA ( Fig. 3a–c ). Following loss of FGF signalling, the expression of runx1 in the DA was expanded beyond the floor region to the roof of the aorta ( Fig. 3d,e ). Cells expressing runx1 were never detected in the surrounding mesenchyme or neighbouring PCV, suggesting that ectopic runx1+ cells must transit through an arterial precursor. Since runx1 is normally expressed only in the aortic floor, the ectopic appearance of runx1+ cells in the aortic roof may indicate that FGF signalling is involved in DA polarization. In mice and zebrafish, DA polarization depends on opposing morphogen gradients; dorsal identity is established by Hedgehog secretion from the notochord, whereas ventral identity relies on BMP production from ventral domains [14] , [15] , [16] . We examined the expression of tbx20 , a transcription factor regulated by Hedgehog signalling [8] , [14] , [51] , which distinguishes the dorsal side of the DA. Neither activation nor inhibition of FGF signalling had any effect on tbx20 expression ( Fig. 3f,h,j ). Examination of transverse sections confirmed that only cells in the roof of the DA and in the developing intersomitic vessels expressed tbx20 , indicating that dorsal polarization is not affected by FGF modulation ( Fig. 3g,i,k,l ). 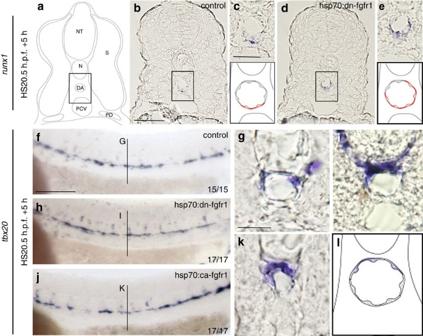Figure 3: Loss of FGF signalling expandsrunx1dorsally without affecting dorsal polarization of the DA. (a) Schematic representation of a trunk section of 26 h.p.f. embryos. (b) Aortic localization ofrunx1+cells in control (b,c) andhsp70:dn-fgfr1(d,e) embryos. Expression oftbx20in control (f,g),hsp70:dn-fgfr1(h,i) andhsp70:ca-fgfr1(j,k) embryos. The black line (G,I,K) denotes where sections were made. (l) Schematic representation oftbx20expression in the roof of the DA. N, notochord; NT, neural tube; PD, pronephric duct; S, somite. Scale bars, 30 μm (b), 200 μm (f) and 20 μm (g). Figure 3: Loss of FGF signalling expands runx1 dorsally without affecting dorsal polarization of the DA. ( a ) Schematic representation of a trunk section of 26 h.p.f. embryos. ( b ) Aortic localization of runx1 + cells in control ( b , c ) and hsp70:dn-fgfr1 ( d , e ) embryos. Expression of tbx20 in control ( f , g ), hsp70:dn-fgfr1 ( h , i ) and hsp70:ca-fgfr1 ( j , k ) embryos. The black line (G,I,K) denotes where sections were made. ( l ) Schematic representation of tbx20 expression in the roof of the DA. N, notochord; NT, neural tube; PD, pronephric duct; S, somite. Scale bars, 30 μm ( b ), 200 μm ( f ) and 20 μm ( g ). Full size image FGF controls HSC formation by modulating BMP activity We next investigated whether FGF regulates the ventral polarization of the DA by modulating BMP activity. In zebrafish, we previously demonstrated that bmp4 is required for the emergence and maintenance of HSCs [14] . Whereas bmp4 is normally expressed in the mesenchyme underlying the DA ( Fig. 4a,d,g ), bmp4 expression was upregulated in the aortic region in the absence of FGF ( Fig. 4b,e,h ). Conversely, in embryos with FGF overactivation, bmp4 was absent from the aortic region ( Fig. 4c,f,i ), supporting the idea that FGF signalling may regulate HSC formation via its effects on the BMP pathway. 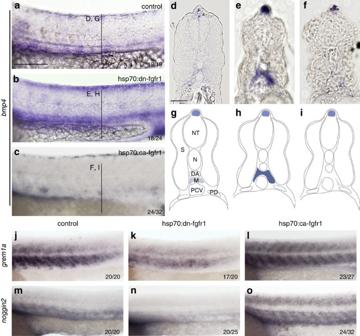Figure 4: FGF signalling regulatesbmp4expression as well asnoggin2andgremlin1a, two BMP antagonists. (a–c)bmp4expression is altered following manipulation of FGF signalling.bmp4levels of expression are increased inhsp70:dn-fgfr1embryos (b,e) and decreased inhsp70:ca-fgfr1embryos (c,f). (d–f) Transverse sections of embryos from WISH samples (a–c). (g–i) Schematic representingbmp4expression in control (g),hsp70:dn-fgfr1(h) andhsp70:ca-fgfr1(i) embryos. (j–o)gremlin1a(j–l) andnoggin2(m–o) expression is reduced inhsp70:dn-fgfr1embryos (k,n) and enhanced inhsp70:ca-fgfr1embryos (l,o). M, mesenchyme. Scale bars, 200 μm (a) and 50 μm (d). Figure 4: FGF signalling regulates bmp4 expression as well as noggin2 and gremlin1a , two BMP antagonists. ( a – c ) bmp4 expression is altered following manipulation of FGF signalling. bmp4 levels of expression are increased in hsp70:dn-fgfr1 embryos ( b , e ) and decreased in hsp70:ca-fgfr1 embryos ( c , f ). ( d – f ) Transverse sections of embryos from WISH samples ( a – c ). ( g – i ) Schematic representing bmp4 expression in control ( g ), hsp70:dn-fgfr1 ( h ) and hsp70:ca-fgfr1 ( i ) embryos. ( j – o ) gremlin1a ( j – l ) and noggin2 ( m – o ) expression is reduced in hsp70:dn-fgfr1 embryos ( k , n ) and enhanced in hsp70:ca-fgfr1 embryos ( l , o ). M, mesenchyme. Scale bars, 200 μm ( a ) and 50 μm ( d ). Full size image Since BMP signalling activity is tightly regulated by several antagonists [52] , we also examined their expression at the time of heat shock. At 20.5 h.p.f., the DA is surrounded by several BMP antagonists, including chordin from the pronephric ducts, as well as noggin1 , noggin2 (ref. 53 ) and gremlin1a [54] . Although chordin is an important regulator of primitive haematopoiesis [55] , it is dispensable for HSC formation [14] . We therefore focused on noggin1 , noggin2 and gremlin1a . In WT embryos, noggin1 is barely detected in the ventral side of the somite at 24 h.p.f., while gremlin1a and noggin2 are strongly expressed in the sclerotome ( Fig. 4j,m ) [53] , [54] . In induced hsp70:dn-fgfr1 embryos, both gremlin1a and noggin2 were markedly downregulated ( Fig. 4k,n ; Supplementary Fig. 6 ). In contrast, when FGF signalling was enforced, there was a substantial upregulation of sclerotomal gremlin1a and noggin2 ( Fig. 4l,o ; Supplementary Fig. 6 ). Augmentation of FGF activity was also observed to induce ectopic expression of gremlin1a and noggin2 in the most dorsal compartment of the somite ( Fig. 4l,o ). Together, these results demonstrate that FGF signalling represses bmp4 expression directly and concomitantly induces expression of the BMP inhibitors noggin2 and gremlin1a in the neighbouring somite. To further analyse how FGF and BMP signalling interact, we tested whether inhibition of BMP signalling in FGF-depleted embryos would affect runx1 expression. Inhibition of FGF signalling, either using the hsp:dn-fgfr1 transgenic animals or a small chemical inhibitor su5402, increases runx1 expression in the DA ( Fig. 5a–c ), while blockage of BMP signalling abrogates runx1 expression ( Fig. 5d ). Inhibition of FGF signalling in a BMP-repressed environment could not rescue HSC production, supporting the idea that FGF acts upstream of the BMP pathway ( Fig. 5e ). 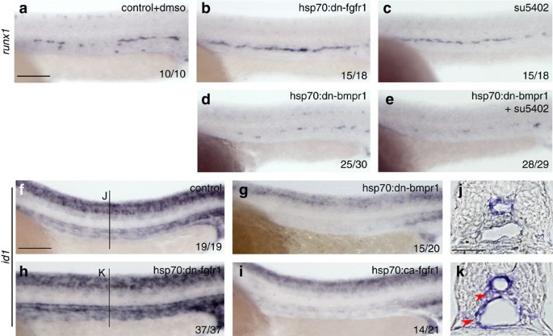Figure 5: Epistatic analysis of BMP and FGF signalling interaction. (a–c)runx1expression is increased inhsp70:dn-fgfr1embryos (b) and embryos treated with su5402 (c) compared with controls (a). Overexpression ofhsp70:dn-bmpr1impairs emergence of HSCs (d) compared with control (a) or FGF-inhibited embryos (b,c). HSC emergence is not rescued inhsp70:dn-bmpr1embryos following blockade of FGF signalling using su5402 (e). (f–k)id1expression is reduced on inhibition of BMP signalling (g) as well as augmentation of FGF signalling (i) compared with control embryos (f). In the absence of FGF signalling,id1expression is increased in the vasculature and in some cells surrounding the vessels (handk, red arrows) compared with control embryos (fandj). Scale bars, 100 μm (a,f) and 30 μm (j). Figure 5: Epistatic analysis of BMP and FGF signalling interaction. ( a – c ) runx1 expression is increased in hsp70:dn-fgfr1 embryos ( b ) and embryos treated with su5402 ( c ) compared with controls ( a ). Overexpression of hsp70:dn-bmpr1 impairs emergence of HSCs ( d ) compared with control ( a ) or FGF-inhibited embryos ( b , c ). HSC emergence is not rescued in hsp70:dn-bmpr1 embryos following blockade of FGF signalling using su5402 ( e ). ( f – k ) id1 expression is reduced on inhibition of BMP signalling ( g ) as well as augmentation of FGF signalling ( i ) compared with control embryos ( f ). In the absence of FGF signalling, id1 expression is increased in the vasculature and in some cells surrounding the vessels ( h and k , red arrows) compared with control embryos ( f and j ). Scale bars, 100 μm ( a , f ) and 30 μm ( j ). Full size image To further examine the epistasis between the FGF and BMP pathways, we sought a molecular marker of BMP activity. The transcriptional repressor id1 is a known target of BMP signalling [56] , and its targeted deletion in the mouse embryo impairs haematopoiesis by affecting the proliferation and the self-renewal of HSCs [57] . In zebrafish, id1 is expressed in developing neural tissue, somites and axial vasculature ( Fig. 5f ); this expression is largely ablated following inhibition of BMP signalling ( Fig. 5g ). Inhibition of FGF signalling leads to an increase in id1 expression in the vasculature ( Fig. 5f,h ), which becomes more apparent in transverse sections ( Fig. 5j,k ). Conversely, stimulation of FGF significantly decreases id1 expression ( Fig. 5i ). Together, these results further demonstrate that the FGF signalling pathway acts upstream of BMP signalling to regulate HSC emergence. Finally, we performed genetic rescue experiments to determine whether enforced BMP signalling could rescue loss of HSCs in hsp70:ca-fgfr1 animals. Enforced activity of the BMP pathway was achieved following induction of a constitutively active bmp receptor 1b ( hse:ca-bmpr1b ) construct in transient transgenic animals, as previously described [58] . Compared with WT siblings, hsp70:ca-fgfr1 animals induced at 20.5 h.p.f. showed loss of HSCs accompanied with an increase in pea3 expression ( Fig. 6a,b,e ). Induction of the hse:ca-bmpr1b transgene alone showed a robust increase in runx1 expression without affecting pea3 ( Fig. 6c,e ). As predicted by our results above, enforced activity of BMP signalling could rescue HSC development in hsp70:ca-fgfr1 animals ( Fig. 6d,e ). 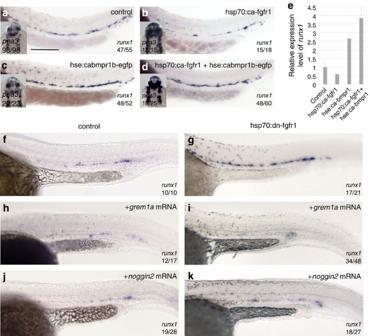Figure 6: Ectopic activation of BMP signalling rescuesrunx1expression in an activated FGF background. (a–d)runx1expression increases in the DA following activation of the BMP pathway (c) compared with controls (a).runx1expression inhsp70:ca-fgfr1(b) embryos is rescued by activation of ahse:ca-bmpr1btransgene (d). Quantitative analysis ofrunx1expression (e). Chart shows results obtained from one representative experiment with three biological replicates (mean±s.d.).pea3expression in the head (inserts,a–d) is upregulated on FGF activation. (f–k)runx1expression is impaired on overexpression of eithergremlin1a(h) ornoggin2(j) compared with control (f). Inhibition of FGF signalling fails to rescuerunx1expression whengremlin1a(i) andnoggin2(k) are overexpressed. Scale bars, 200 μm (a). Figure 6: Ectopic activation of BMP signalling rescues runx1 expression in an activated FGF background. ( a – d ) runx1 expression increases in the DA following activation of the BMP pathway ( c ) compared with controls ( a ). runx1 expression in hsp70:ca-fgfr1 ( b ) embryos is rescued by activation of a hse:ca-bmpr1b transgene ( d ). Quantitative analysis of runx1 expression ( e ). Chart shows results obtained from one representative experiment with three biological replicates (mean±s.d.). pea3 expression in the head (inserts, a – d ) is upregulated on FGF activation. ( f – k ) runx1 expression is impaired on overexpression of either gremlin1a ( h ) or noggin2 ( j ) compared with control ( f ). Inhibition of FGF signalling fails to rescue runx1 expression when gremlin1a ( i ) and noggin2 ( k ) are overexpressed. Scale bars, 200 μm ( a ). Full size image In this experiment, BMP signalling was enforced at the receptor level, bypassing therefore any potential effect of the Bmp antagonists noggin2 and gremlin1a. In hsp:ca-fgfr1 embryos, their expression levels are elevated suggesting that they may reinforce the BMP-repressive environment in the DA. According to this hypothesis, overexpression of noggin2 or gremlin1a following inhibition of FGF signalling should prevent runx1 increase. Overexpressions of noggin2 and gremlin1a were achieved by mRNA injection into hsp70:dn-fgfr1 embryos and analysed for runx1 expression. As predicted, both noggin2 and gremlin1a repress HSC formation when injected in control embryos ( Fig. 6f,h,j ). Similar results were obtained when noggin2 and gremlin1a were overexpressed in hsp:dn-fgfr1 embryos ( Fig. 6g,i,k ), confirming that both antagonists are acting downstream of FGF signalling and upstream of bmp4/bmpr1. Collectively, our results indicate that FGF signalling controls the emergence of HSCs by modulating the activity of BMP signalling in the aortic region. The inhibition of BMP signalling by FGF acts at two levels, first by repressing the transcription of bmp4 in the subaortic mesenchyme and second by increasing the expression of BMP antagonists in the neighbouring somite. These results suggest that the level of FGF signalling controls the capacity of the aortic microenvironment to support or repress the formation of HSCs ( Fig. 7 ). 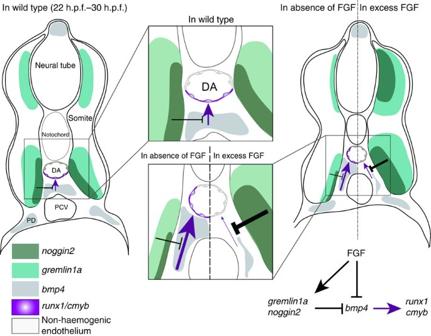Figure 7: Role of FGF signalling in the formation of HSCs. Model for the regulation of HSC emergence by FGF signalling. Figure 7: Role of FGF signalling in the formation of HSCs. Model for the regulation of HSC emergence by FGF signalling. Full size image Despite FGF signalling playing key roles in the formation of mesoderm and the vascular system, no previous studies have examined potential roles for FGF in HSC development. Studies in adult mice have demonstrated that HSCs express Fgfr1, and that provision of Fgf1 ex vivo can stimulate HSC expansion [27] . More recent work, however, has demonstrated that Fgfr1 is not required for the normal homeostasis of adult HSCs, but rather in haematopoietic recovery following injury via irradiation or chemotherapy by stimulating HSC proliferation [30] . FGF signalling may therefore be important in regulating the number of adult HSCs. A current bottleneck in the field of regenerative medicine is the inability to instruct HSC fate in vitro from pluripotent precursors, including induced pluripotent stem cells. This is due, at least in part, to an incomplete understanding of the native factors that are required to specify HSCs during embryonic development. In this study, we have demonstrated a novel requirement for FGF signalling in the generation of HSCs. We show that FGF represses the emergence and maintenance of HSCs in the DA by blocking BMP signals that originate from the aortic mesenchyme. This negative role is in contrast to the role that FGF signalling has in adult haematopoiesis, where it promotes HSC amplification. Along with the results of the companion paper (Lee et al . ), it is now apparent that the FGF pathway is required at multiple stages of development to properly specify HSC fate. HSCs originate from arterial precursors, which depend on the Notch and Vegf signalling pathways for their specification and differentiation [7] , [9] , [11] , [21] , [48] , [49] , [59] . Unlike the results of Lee et al ., where early FGF signalling (14–17 h.p.f.) is required within the somite to bridge the Wnt16-mediated expression of the Notch ligand deltaC , the subsequent FGF signalling requirement (22–30 h.p.f.) for HSC emergence lies downstream of Notch function. Neither Notch- nor Vegf-dependent gene expression programmes were affected following modulation of FGF activity after 20.5 h.p.f. Moreover, the combined inhibition of Notch and FGF signalling failed to decrease runx1 expression in the DA, indicating that FGF acts downstream of the Notch pathway in HSC emergence. Interestingly, while FGF inhibition increased the number of HSCs emerging from the DA, we did not observe ectopic runx1 + cells outside of the DA, suggesting that FGF signalling affects only arterial precursors previously specified by Notch signalling. Following the induced repression of FGF signalling, runx1 expression expands dorsally within the DA without affecting dorsal identity, as defined by the normal expression of tbx20 . This finding suggests that the expression domains of runx1 and tbx20 are not mutually exclusive, confirming our previous report [14] . Interestingly, the expanded pool of runx1+/cmyb+ cells behave as normal HSC. Ectopically induced HSCs have the capacity to migrate from the DA, seed the different haematopoietic organs and differentiate into T cells in the embryos showing normal blood flow 2 to 3 days after heat shock. The proper establishment of ventral aortic identity, in contrast to the dorsal identity, appears to depend on the FGF pathway. FGF signalling controls the ventral polarization of the DA by restricting bmp4 expression in the mesenchyme around the aortic endothelium. The timing and location of bmp4 expression in the subaortic mesenchyme is conserved among several classes of vertebrates [14] , [15] , [17] , [60] . Interestingly, clusters of blood cells emerge from both the dorsal and ventral side of the DA in mouse embryos [61] . However, the adult reconstituting potential is restricted to the ventral clusters [62] , supporting the idea that the ventral mesenchyme provides the cues critical to conferring stem cell potential. This hypothesis is supported by previous findings, where early resection of ventral mesenchyme led to loss of aortic runx1 expression and haematopoietic cluster formation [3] . Our analysis of fgfr2 and fgfr3 expression patterns showed that, while fgfr3 is mainly found in the somitic tissue at the time of HSC emergence, fgfr2 transcripts are detected in the few cells surrounding the axial vasculature corresponding to the territory of expression of bmp4 . This tissue localization suggests that fgfr2 may mediate the effect observed on bmp4 expression when FGF signalling is modulated. Fgf10a, whose loss gives rise to a similar haematopoietic phenotype to that observed in the hsp:dn-fgfr1 , was shown to preferentially interact with fgfr2 (ref. 63 ), supporting the existence of an axis involving fgf10a/fgfr2/bmp4 to play the role of a switch that triggers the aortic blood programme. However, we cannot rule out that other Fgf ligands may be involved in the regulation of HSC specification from the haemogenic endothelium. Our attempts to mimic the hsp70:dn-fgfr1 phenotype by knocking down fgfr2 and fgfr3 failed and morphant embryos showed a drastic decrease in runx1 expression at 26 h.p.f. Knowing that Fgf receptors can heterodimerize [64] and that both fgfr2 and fgfr3 are expressed early in the forming somites [65] , [66] , it is possible that fgfr2 and fgfr3 may be required in the somites to promote HSC specification in concert with fgfr1 and fgfr4 . To better understand how and when each receptor mediates the activity of the FGF signalling, new tools offering time control and tissue specificity have to be developed. Our previous studies demonstrated that bmp4 is crucial for HSC formation in zebrafish [14] . Attempts to locally increase Bmp4 activity using the zebrafish mutant in chordin , a Bmp antagonist, failed to increase runx1 expression in the DA [14] , suggesting that bmp4 alone is insufficient for HSC formation or that other Bmp antagonists regulate HSC emergence. Our current findings indicate that the regulation of BMP signalling by FGF acts at multiple levels. First, enforced expression of a constitutively active Bmp receptor 1 rescued runx1 expression in hsp70:ca-fgfr1 embryos, indicating that BMP signalling is sufficient to trigger the definitive haematopoietic programme in the DA. This result, along with the finding that combined inhibition of FGF and BMP failed to generate HSCs, indicates that FGF signalling acts genetically upstream of BMP. In addition, inhibition of FGF function substantially increases bmp4 expression in the subaortic mesenchyme and prevents expression of two BMP antagonists, noggin2 and gremlin1a , in the surrounding somites. Here we report that overexpression of either noggin2 or gremlin1a is enough to prevent runx1 upregulation in the absence of FGF. This indicates that local increases in bmp4 should be accompanied by inhibition of the bmp4 antagonists, gremlin1a and noggin2 , to trigger the definitive blood programme. Collectively, these results indicate that ablation of FGF signalling intensifies the effects of BMP signalling in the DA on the haematopoietic programme by both enhancing the expression of bmp4 directly and repressing the expression of local BMP antagonists. In conclusion, we show that the FGF signalling pathway is a negative regulator of HSC emergence through its control of bmp4 function underlying the aortic floor. FGF signalling may thus provide a missing link in what regulates the developmental switch from a BMP repressive to supportive environment that is linked to the emergence of HSCs from ventral aortic endothelium. These findings suggest that careful modulation of the FGF/BMP signalling axis may be important in the instruction of HSC fate in regenerative medicine approaches. Zebrafish strains WT AB* and transgenic lines, hsp70:dn-fgfr1 (Tg( hsp70l:dnfgfr-EGFP) pd1 ) [33] , hsp70:ca-fgfr1 (Tg( hsp70l:Xla.fgfr1, cryaa:DsRed ) pd3 ) [34] and hsp70:dn-bmpr1 tg(hsp70l:dn-bmpr1-EGFP) [67] , were maintained and stage as previously described in ref. 68 . All animal work was carried out according to UK Home Office and UCSD IACUC regulations and under the appropriate project license. Heat-shock conditions Embryos were heat shocked by transferring them into prewarm E3 medium for 30 min at either 39 °C for hsp70:dn-fgfr1 , hsp70:ca-fgfr1 and hsp70:ca-fgfr1 injected with HSE:ca-bmpr1b-EGFP construct [58] or 43 °C for hsp70:dn - bmpr1 , then transferred to 28 °C until fixation. Transgenic embryos were selected based on their reporter expression or by genotyping as previously described in ref. 69 . After in situ hybridization, embryos were subdissected. Single heads were incubated for 60 min at 95 °C in lysis buffer (25 mM NaOH, 0.2 mM EDTA), samples were then buffered with 40 mM Tris-HCl, pH 8. Genomic DNA was used for PCR amplification to detect DsRed transgene using forward 5′- CATCCTGTCCCCCCAGTTCC -3′ and reverse 5′- CCCAGCCCATAGTCTTCTTCTGC -3′ primers (255-base-pair product). Chemical treatments Small-molecule inhibitors were resuspended in dimethylsulphoxide (DMSO) and diluted in E3 medium. Su5402 (Calbiochem) was used at 5 μM and DAPM (Calbiochem) at 100 μM (ref. 70 ). Control embryos were treated with the corresponding volumes of DMSO added to E3 medium just after heat shock. WISH Embryos were fixed in fresh paraformaldehyde 4%, dehydrated in EtOH and assayed for WISH as described in ref. 8 . RNA probes were labelled with digoxigenin (Roche) and detected using an anti-Dig antibody (1/5,000, Roche). Embryos were stained using a solution of NBT/BCIP (nitro-blue tetrazolium/5-bromo-4-chloro-3-indolylphosphate p-toluidine salt) (Roche). Wax sectioning Embryos were dehydrated in EtOH 100% overnight, transferred into xylene for 30 min and then embedded in wax. Blocks containing stained embryos were sectioned at 10 or 4 μm using a microtome (Leica). Sections were transferred onto glass slides, incubated at 37 °C overnight. Wax was removed in xylene and EtOH 100, 70 and 50%, and rehydrated in PBS. Slides were mounted and imaged. For the Fgf receptors, representative embryos were selected and transversally sectioned using a razor blade. Slices of embryos were then soaked in glycerol and imaged. Transient transgenesis and injection experiments 20 pg of HSE:ca-bmpr1b-EGFP transgenesis construct [58] combined with 25 pg of transposase mRNA was injected in one-cell stage of AB* or hsp70:ca-fgfr1 embryos. As a negative control, the construct was injected without transposase. One-cell stage embryos were injected with morpholino solution diluted in water. Injected and uninjected embryos were incubated at 28 °C until fixation. Sequences and working concentrations are available in Supplementary Table 1 . Real-time PCR Total RNA was isolated from dissected trunk embryos 5 h after heat shock using the RNAeasy Micro Kit (Qiagen). Single heads of hsp70:ca-fgfr1 were used for genotyping, while corresponding trunks were kept individually on dry ice. Positive trunks were then pooled and processed as other samples with Superscript III Reverse Transcriptase (Invitrogen). qPCR was performed with Sybr Green (Applied Biosystems) and analysed by the comparative method (ΔΔ C t ) with ef1α housekeeping gene as internal control. Statistical analysis was performed using t -test. Primer sequences available in Supplementary Table 1 . Statistical analysis All the experiments presented in this study were performed at least three times. Data were collected from independent experiments and are given as the mean±s.d. Student’s t -test was used for statistical comparisons and P< 0.05 was considered statistically significant. How to cite this article: Pouget, C. et al . FGF signalling restricts haematopoietic stem cell specification via modulation of the BMP pathway. Nat. Commun. 5:5588 doi: 10.1038/ncomms6588 (2014).